The crystal structure of multidrug-resistance regulator RamR with multiple drugs RamR is a transcriptional repressor of the gene-encoding RamA protein, which controls the expression of the multidrug efflux system genes acrAB-tolC . RamR is an important multidrug-resistance factor, however, its structure and the identity of the molecules to which it responds have been unknown. Here, we report the crystal structure of RamR in complex with multiple drugs, including berberine, crystal violet, dequalinium, ethidium bromide and rhodamine 6G. All compounds are found to interact with Phe155 of RamR, and each compound is surrounded by different amino acid residues. Binding of these compounds to RamR reduces its DNA-binding affinity, which results in the increased expression of ramA . Our results reveal significant flexibility in the substrate-recognition region of RamR, which regulates the bacterial efflux participating in multidrug resistance. The increasing prevalence of multiple drug resistance in pathogenic bacteria is a major threat to human health. Bacterial multidrug resistance can be defined as the ability of bacteria to survive lethal doses of structurally diverse drugs that are able to eradicate non-resistant cells. One important mechanism that gives rise to multidrug resistance is the active efflux of drugs by multidrug transporters. The important role of drug efflux systems in multidrug resistance has been well documented in eukaryotes as well as in prokaryotes [1] , [2] . Gram-negative bacteria are often intrinsically resistant to a number of antimicrobial agents, and multidrug transporters of the resistance-nodulation-cell division family such as AcrAB are particularly effective in generating this resistance [3] . In bacteria, transcriptional activators and/or repressors tightly regulate the expression of a number of multidrug transporter genes. The transcriptional regulation of these transport systems is achieved by local regulators, which are encoded in the same gene clusters as efflux transporters and by global regulators, which are encoded in other genomic regions and whose regulatory action can also affect functions other than multidrug resistance [4] , [5] , [6] , [7] . Regulation of resistance-nodulation-cell division multidrug transporters has been widely studied in Escherichia coli . For example, acrAB expression is modulated by the local repressor AcrR, and by the global regulators MarA, SoxS and Rob, which belong to the AraC/XylS family of transcriptional regulators [8] . In several pathogens, including Salmonella spp., Enterobacter aerogenes , Enterobacter cloacae and Klebsiella pneumoniae , the RamA global transcriptional activator, which belongs to the AraC/XylS family of regulatory proteins, participates in multidrug resistance by activating the expression of AcrAB [9] , [10] , [11] , [12] . RamA has also been reported to negatively influence virulence in Salmonella enterica serovar Typhimurium by downregulating SPI-1 expression [13] . However, this seems to be dependent on the genetic background of the strain [14] . Abouzeed et al. [15] identified the ramR gene, which is located directly upstream of ramA and encodes a protein of the TetR family of transcriptional repressors ( Fig. 1a ). Its role as a local repressor of ramA was determined by inactivation and complementation experiments [15] . RamR binds to the region upstream of ramA . Its binding site covers essential features of the ramA promoter, including the −10 conserved region, the transcriptional start site of ramA and two 7-bp inverted repeats [16] . Various types of mutations in ramR and the ramR–ramA intergenic region were identified in multidrug-resistant strains of S . typhimurium , other S. enterica serovars and K. pneumoniae , which result in increased expression of ramA and an increase in efflux-mediated multidrug resistance [15] , [17] , [18] . 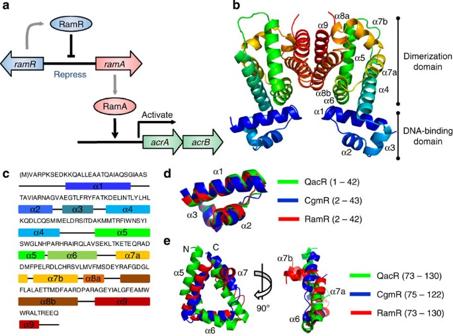Figure 1: Regulatory cascade and structure of RamR. (a) Model for gene regulation by RamR. RamR represses theramAgene, which encodes the activator protein for theacrABdrug efflux pump genes. RamR binds to the intergenic region between theramRandramAgenes, and RamA binds to the upstream region toacrAB. (b) Crystal structure of the RamR dimer. Each monomer is coloured as follows: the α-helices are represented in blue (α1), marine (α2), sky blue (α3), cyan (α4), green (α5), limon (α6), yellow (α7a), deep olive (α7b), orange (α8a), brown (α8b) and red (α9). (c) Secondary structure elements and amino acid sequence of the RamR protomer. RamR composes of nine α-helices (α1–α9). Because α7 and α8 are tortuous, they are subdivided into regions denoted α7a, α7b, α8a and α8b based on the borders of this tortuosity. Each of α-helices are coloured according to the scheme used inb. (d) Structures of DNA-binding sites of QacR, CgmR and RamR. Helices α1, α2 and α3 of QacR (amino acids 1–42) are represented in green, of CgmR (2–43) in blue and of RamR (2–42) in red. (e) Structures of the C-termini of TetR family regulators. Structures of helices α5, α6 and α7 of QacR (amino acids 73–130) are represented in green, of CgmR (75–122) in blue and of RamR (73–130) in red. Because α7 of RamR is tortuous, its shape is different from those of QacR and CgmR. Figure 1: Regulatory cascade and structure of RamR. ( a ) Model for gene regulation by RamR. RamR represses the ramA gene, which encodes the activator protein for the acrAB drug efflux pump genes. RamR binds to the intergenic region between the ramR and ramA genes, and RamA binds to the upstream region to acrAB . ( b ) Crystal structure of the RamR dimer. Each monomer is coloured as follows: the α-helices are represented in blue (α1), marine (α2), sky blue (α3), cyan (α4), green (α5), limon (α6), yellow (α7a), deep olive (α7b), orange (α8a), brown (α8b) and red (α9). ( c ) Secondary structure elements and amino acid sequence of the RamR protomer. RamR composes of nine α-helices (α1–α9). Because α7 and α8 are tortuous, they are subdivided into regions denoted α7a, α7b, α8a and α8b based on the borders of this tortuosity. Each of α-helices are coloured according to the scheme used in b . ( d ) Structures of DNA-binding sites of QacR, CgmR and RamR. Helices α1, α2 and α3 of QacR (amino acids 1–42) are represented in green, of CgmR (2–43) in blue and of RamR (2–42) in red. ( e ) Structures of the C-termini of TetR family regulators. Structures of helices α5, α6 and α7 of QacR (amino acids 73–130) are represented in green, of CgmR (75–122) in blue and of RamR (73–130) in red. Because α7 of RamR is tortuous, its shape is different from those of QacR and CgmR. Full size image The regulators usually bind many of the same structurally and chemically diverse drugs that are effluxed by the transporters that they regulate. Therefore, these regulators act as cytosolic multidrug sensors that respond to threatening amounts of drug as they overwhelm the multidrug transporters. Although it is an important regulator of multidrug resistance in several pathogens, the structure of RamR and the drugs to which this regulatory protein binds have not been reported yet. Here we report the crystal structure of RamR in complex with multiple drugs. All of the compounds tested were found to interact with RamR resulting in a decreased DNA-binding affinity, and consecutive increased expression of ramA . Structure of the RamR protein The molecular weight of RamR in solution was calculated to be 36 kDa using gel filtration chromatography, which was conducted during the purification of the RamR protein ( Supplementary Fig. S1 ). Dissolved RamR was found to exist in the dimer form in solution, and the molecular weight of the RamR monomer was 21 kDa. The structure of RamR was initially determined at a resolution of 2.6 Å by multiple wavelength anomalous dispersion using selenomethionine modification ( Supplementary Table S1 ). Subsequently, we determined the RamR structure at 2.1 Å by molecular replacement ( Fig. 1b and Supplementary Table S1 ). Approximate overall dimensions of the RamR dimer were 58 × 47 × 44 Å (ref. 3 ) (corresponding to the width, height and depth of the molecule in the orientation shown in Fig. 1b ). All polypeptide chains (residue numbers 8–191) were helical and composed of nine α-helices (α1–α9) ( Fig. 1c ). The three-helix bundle structures formed at the RamR N-terminus (α1–α3) maintained a helix-turn-helix motif conserved in DNA-binding sites. The structure of the RamR DNA-binding site is similar to that of other TetR family regulators ( Fig. 1d ). The C-terminus of RamR is composed of six α-helices, which include important regions for dimerization. Dimerization occurs through hydrogen bonding and hydrophobic interactions in α8–α9 ( Fig. 1b ). In addition, α4–α9 was observed to consist of a six-helix bundle structure, and RamR may recognize a substrate in this region. It was previously suggested that the central triangle (α5–α7) is conserved in the C-terminus structure of TetR family regulators [19] . However, we found that this central triangle was not conserved in RamR because of its tortuosity in α7 ( Fig. 1e ). Although a loop structure is evident in the junction between α7 and α8 in other TetR family regulators, this junction is represented by an α-helix in RamR. This may be a reason that the central triangle was not conserved in RamR. Induction of RamR regulon by multiple drugs Because RamR has a putative substrate-recognition site, it was hypothesized that some chemical compounds might bind to this protein. To identify chemical compounds that bind to RamR, we employed surface plasmon resonance (SPR) analysis using a Biacore T200 (GE Healthcare). We tested individual solutions of several compounds (chloramphenicol, crystal violet, dequalinium, erythromycin, ethidium bromide, oxacillin, rhodamine 6G, rifampicin, tetracycline and trimethoprim), including AcrAB substrates, which were separately run over RamR immobilized on a CM5 sensor chip. We found that five compounds, berberine, crystal violet, dequalinium, ethidium bromide and rhodamine 6G ( Fig. 2a ), bind to the RamR protein ( Supplementary Fig. S2 ). The SPR responses indicated that all compounds directly bound to RamR, and the responses increased in a concentration-dependent manner (0.31–20 μM). In contrast, tetracycline did not show any indication of binding to RamR at concentrations up to 20 μM. K D values of berberine, crystal violet, dequalinium, ethidium bromide and rhodamine 6G, calculated from SPR data, were 17.9±0.03, 21.2±0.53, 21.2±0.42, 14.6±0.10 and 26.4±0.08 μM, respectively. 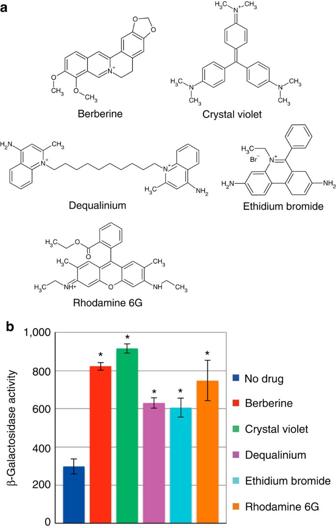Figure 2: Drugs that induce the RamR-regulated generamA. (a) The chemical structures of five compounds: berberine, crystal violet, dequalinium, ethidium bromide and rhodamine 6G that were found to bind to the RamR protein from the SPR analysis (Supplementary Fig. S2). (b) Effect of drugs onramAtranscription. β-Galactosidase levels were assayed in the wild-type strain carrying theramAreporter plasmid (pNNramA) (NES84). Cells were grown in LB supplemented with 2 mM ethidium bromide, 0.1 mM dequalinium, 1 mM rhodamine 6G and 0.2 mM crystal violet or 2 mM berberine. The values displayed correspond to the mean of three independent experiments. Bars correspond to the s.d. Student’st-test; *,P<0.01 versus control. Figure 2: Drugs that induce the RamR-regulated gene ramA . ( a ) The chemical structures of five compounds: berberine, crystal violet, dequalinium, ethidium bromide and rhodamine 6G that were found to bind to the RamR protein from the SPR analysis ( Supplementary Fig. S2 ). ( b ) Effect of drugs on ramA transcription. β-Galactosidase levels were assayed in the wild-type strain carrying the ramA reporter plasmid (pNN ramA ) (NES84). Cells were grown in LB supplemented with 2 mM ethidium bromide, 0.1 mM dequalinium, 1 mM rhodamine 6G and 0.2 mM crystal violet or 2 mM berberine. The values displayed correspond to the mean of three independent experiments. Bars correspond to the s.d. Student’s t -test; *, P <0.01 versus control. Full size image On the basis of these results, it was suggested that these compounds may influence the expression level of ramA . To confirm this possibility, we tested the effect of these RamR ligands on the promoter activity of ramA . Using a ramA reporter plasmid, a β-galactosidase assay showed the enhanced promoter activity of ramA when bacterial cells were treated with berberine (2.7-fold increase), crystal violet (3.1-fold increase), dequalinium (2.1-fold increase), ethidium bromide (2.0-fold increase) or rhodamine 6G (2.5-fold increase) ( Fig. 2b ). Co-crystal structures of RamR with multiple drugs Based on the structure of drug-free RamR, we hypothesized that this protein has a ligand-binding pocket formed by the C-terminal domain. According to our SPR analysis, multiple compounds may interact with this putative ligand-binding pocket. To demonstrate the existence of the C-terminal domain-binding pocket, we needed to determine the structures of the RamR substrate complexes. Therefore, we determined the crystal structures of RamR in complex with berberine, crystal violet, dequalinium, ethidium bromide and rhodamine 6G ( Fig. 3 ). Electron density maps of each co-crystal structure are shown in Supplementary Fig. S3 . The crystal structures were refined to a resolution of 2.4 Å, 2.2 Å, 2.6 Å, 1.6 Å and 2.5 Å, respectively ( Supplementary Table S2 ). The structure reveals that RamR binds two molecules of berberine, ethidium bromide or rhodamine 6G per dimer. And RamR binds one crystal violet or dequalinium molecule per dimer. It was originally reported that all the ligands bind to QacR with a 1:2 stoichiometry (one ligand per QacR dimer), [20] whereas either 1:2 or 1:1 stoichiometry has been observed for RamR. Similar observations were reported in TtgR [21] . All the drugs studied, except dequalinium, were found completely buried in the RamR-binding pocket. Most of the dequalinium is buried in the binding pocket; however, one of the two aromatic rings in both the sides of this compound exists outside the pocket because dequalinium is longer than the other compounds ( Fig. 2a ). The orientation of all drugs is parallel with the Phe155 of RamR, suggesting that all these drugs bind with RamR through π–π stacking interactions. In contrast to the common interaction of all of these drugs with Phe155, each individual drug was also found to interact with a different set of amino acid residues other than Phe155 ( Supplementary Table S3 ). The interaction of different sets of amino acid residues with each drug indicates that multiple drugs are recognized by the multisite binding of RamR. 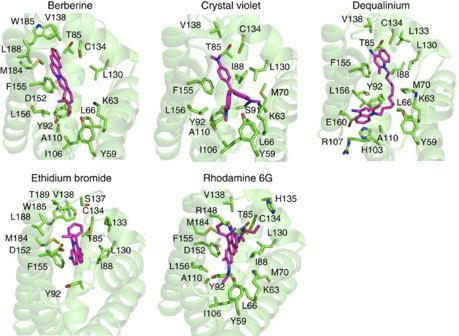Figure 3: Multidrug recognition by RamR. Substrate-binding site of RamR with a bound molecule berberine, crystal violet, dequalinium, ethidium bromide or rhodamine 6G. Key residues are shown, including residue Phe155, which is involved in π–π stacking interactions with drugs. Carbon atoms of drugs and RamR are shown in magenta and green, respectively. Nitrogen, oxygen and sulphur atoms are shown in blue, red and yellow, respectively. Figure 3: Multidrug recognition by RamR. Substrate-binding site of RamR with a bound molecule berberine, crystal violet, dequalinium, ethidium bromide or rhodamine 6G. Key residues are shown, including residue Phe155, which is involved in π–π stacking interactions with drugs. Carbon atoms of drugs and RamR are shown in magenta and green, respectively. Nitrogen, oxygen and sulphur atoms are shown in blue, red and yellow, respectively. Full size image Comparison of the liganded structures with an unliganded RamR structure determined in our lab ( Supplementary Fig. S4 ) reveals that drug binding triggers an expansion of the distance between the N-termini of the helix-turn-helix motifs in the RamR dimer. This expansion occurred as a result of the binding of all the drugs we examined. The average expansion of the distance between the α-carbons of amino acid residues 9 and 50 are 5.9 Å (berberine), 5.1 Å (crystal violet), 8.4 Å (dequalinium), 5.6 Å (ethidium bromide) and 6.0 Å (rhodamine 6G). This movement may contribute to the reduction in RamR DNA-binding affinity required to derepress ramA expression in response to multiple drugs. Reduction of DNA-binding affinity of RamR by multiple drugs Bacterial multidrug efflux regulators usually control the expression of multidrug efflux pumps by binding to inverted repeat sequences in their promoter regions. A recent study using footprinting analysis revealed the 28-bp RamR-binding site [16] . On the basis of the RamR footprint and electrophoretic mobility shift assays (EMSAs), it was proposed that RamR interacts with P ramA as a dimer of dimers [16] . Our results suggest that the binding of multiple drugs to RamR may reduce its DNA-binding affinity, resulting in the induction of ramA expression. To test this hypothesis, EMSA was performed with purified RamR protein and a 100-bp DNA fragment containing the RamR-binding site. These experiments were performed in the absence or presence of drugs that are substrates of the AcrAB efflux system and are found to be bound to the RamR protein. Tetracycline was used in this assay as a negative control. As shown in Fig. 4a , the shift of the DNA band was dependent on the protein concentration [16] . Addition of berberine, crystal violet, dequalinium, ethidium bromide or rhodamine 6G to the RamR–DNA complex resulted in the loss of the retarded band, indicating the separation of the protein and DNA components. In contrast to these compounds, tetracycline did not affect the retarded band because tetracycline did not bind to RamR as mentioned before. 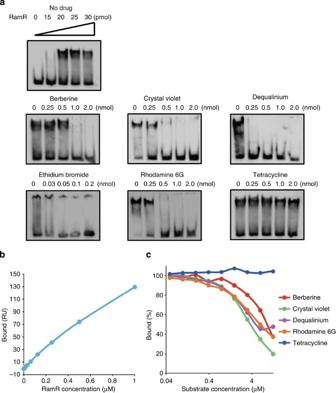Figure 4: Inhibitory effects of drugs on the DNA-affinity of RamR. (a) EMSA for RamR binding to DNA. The labelled DNA (15.5 fmol) was incubated with increasing concentrations (0, 15, 20, 25 or 30 pmol) of the purified RamR protein (upper left). To test the inhibitory effect of berberine, crystal violet, dequalinium, ethidium bromide and rhodamine 6G on DNA–RamR binding, each drug was added to an incubation mixture containing the labelled DNA and 20 pmol RamR, at the concentrations indicated. Tetracycline was used as a negative control. (b) Binding of RamR to DNA analysed by SPR. DNA was immobilized onto a sensor chip, and then purified RamR protein was injected at different concentrations as indicated. (c) Inhibitory effects of drugs on RamR and DNA binding calculated from the results of SPR analysis. DNA was immobilized onto a sensor chip, and then the purified RamR protein (2 μM) was run over the sensor surface in the presence or absence of drugs at the various concentrations indicated. Percentage bound was calculated from the amount of RamR binding with DNA in the absence of drug, which was assigned as 100%. Shown is the result of one of the three experiments, which gave similar results. Figure 4: Inhibitory effects of drugs on the DNA-affinity of RamR. ( a ) EMSA for RamR binding to DNA. The labelled DNA (15.5 fmol) was incubated with increasing concentrations (0, 15, 20, 25 or 30 pmol) of the purified RamR protein (upper left). To test the inhibitory effect of berberine, crystal violet, dequalinium, ethidium bromide and rhodamine 6G on DNA–RamR binding, each drug was added to an incubation mixture containing the labelled DNA and 20 pmol RamR, at the concentrations indicated. Tetracycline was used as a negative control. ( b ) Binding of RamR to DNA analysed by SPR. DNA was immobilized onto a sensor chip, and then purified RamR protein was injected at different concentrations as indicated. ( c ) Inhibitory effects of drugs on RamR and DNA binding calculated from the results of SPR analysis. DNA was immobilized onto a sensor chip, and then the purified RamR protein (2 μM) was run over the sensor surface in the presence or absence of drugs at the various concentrations indicated. Percentage bound was calculated from the amount of RamR binding with DNA in the absence of drug, which was assigned as 100%. Shown is the result of one of the three experiments, which gave similar results. Full size image We also conducted SPR experiments using the 100-bp DNA fragment and the RamR protein to quantify the effects of RamR substrates on the RamR interaction with its DNA-binding site. A solution of RamR protein was run over the DNA fragment immobilized on a sensor chip SA, in the presence or absence of drugs. RamR bound to DNA in a concentration-dependent manner ( Fig. 4b ) and berberine, crystal violet, dequalinium and rhodamine 6G inhibited the binding of RamR to the DNA fragment containing its binding site, whereas tetracycline did not ( Fig. 4c ). In case of ethidium bromide, there was a lot of noise because of the affinity of ethidium bromide to DNA. Therefore, it was difficult to see its inhibitory effect on the binding of RamR to the immobilized DNA. These experiments revealed that RamR substrates interact with their recognition sites to reduce the DNA-binding affinity of RamR, resulting in the induction of ramA . We report a multidrug-recognition mechanism of RamR, whereby the DNA-binding activity is controlled by multiple drugs to induce ramA expression. Determining the crystal structure of RamR is the first step in understanding the structural basis for the function of the regulatory proteins that control both drug resistance and virulence in pathogens. In this study, we identified five substrates of the RamR protein, including berberine, crystal violet, dequalinium, ethidium bromide and rhodamine 6G. Similar approaches in crystallizing the TetR family regulators with multiple drugs have been also reported in QacR [20] , TtgR [21] and CmeR [22] . Our knowledge should advance efforts aimed at identifying small molecules that could modulate the function of the RamR protein. RamR is an important factor of multidrug resistance because recent studies identified mutations in RamR in multidrug-resistant clinical isolates, including S. enterica and K. pneumoniae . Previous studies have identified six amino acid substitutions in RamR that are related to bacterial drug resistance, including T18P, R46N, R46P, Y59H, M84I and E160D [15] , [17] , [23] . As shown in Supplementary Fig. S5 , T18 and R46 exist in the DNA-binding domain. Thus, amino acid substitutions at these positions might destroy the structure of the DNA-binding domain, resulting in the reduction of its DNA-binding affinity. Amino acid residues Y59 and E160 are considered to be involved in RamR substrate recognition ( Supplementary Table S3 ), and M84 is adjacent to M85, which is suggested to be an important residue in the recognition of all five drugs ( Supplementary Table S3 ). Thus, amino acid substitutions at positions Y59, M84 and E160 might expand the distance between the N-termini of the helix-turn-helix motifs in the RamR dimer. This may reduce the DNA-binding affinity of RamR, resulting in increased expression levels of ramA and acrAB . In conclusion, we have made an effort to extend our knowledge of transcriptional regulation mediated by RamR, a regulator of multidrug resistance in several enterobacterial pathogens. Bacterial strains and plasmids The bacterial strains and plasmids used in this study are listed in Supplementary Table S4 . S. enterica serovar Typhimurium strains used in this study were the wild-type strain ATCC14028s [24] and its derivatives. Growth conditions Bacterial strains were grown at 37 °C in Luria Bertani (LB) broth supplemented with ampicillin (100 μg ml −1 ), kanamycin (25 μg ml −1 ) or chloramphenicol (25 μg ml −1 ) where appropriate. Protein preparation The ramR gene was amplified by PCR from the genomic DNA of strain ATCC14028s using primers ramR -F- Nco I and ramR -R- Bgl II ( Supplementary Table S5 ). The PCR product was digested with Nco I and Hin dIII and then cloned into the pETDuet-1 vector. The E. coli C41 (DE3) strain was transformed with pETDuet-1, and the transformant was grown at 37 °C in LB containing ampicillin (100 μg ml −1 ). Isopropyl β- D -1-thiogalactopyranoside was added to induce the protein production in the bacterial culture with an optical density of 0.6 at 600 nm. Subsequently, cultures were incubated for 3 h, cells were collected by centrifugation and the pellet was suspended in a buffer (50 mM sodium phosphate (pH 7.0), 1 mM EDTA and 1 mM dithiothreitol (DTT)). After the cells were disrupted using a French Pressure Cell (SLM Aminco), RamR was purified using a two-step procedure. Cation exchange chromatography using SP-Sepharose FF (GE Healthcare) was followed by gel filtration on a Superdex 200 10/300 GL column (GE Healthcare) and eluted with buffer containing 20 mM Tris (pH 8.0), 200 mM NaCl and 3 mM DTT. Crystallization and data collection Crystals were grown from hanging drops at 25 °C using the vapour diffusion method. To form co-crystals of RamR with drugs, substrates were added to the purified protein and incubated overnight. Protein solution contained 20 mM Tris (pH 8.0), 75 mM KCl, 2 mM DTT (for unliganded RamR) or 20 mM sodium phosphate (pH 6.6), 75 mM NaCl and 2 mM DTT (for liganded RamR). The crystals grew to optimal size within 1 week. The crystals were cryoprotected using a solution containing PEG200 (for unliganded RamR) or 25% glycerol (for co-crystals of RamR with substrates). Crystals were picked using nylon loops (Hamoton Research) and subjected to flash cooling in cold nitrogen gas from a cryostat (Rigaku). All data sets were collected on beamline BL44XU at SPring-8 with a charge-coupled device detector Quantum 315 (ADSC) and imaging-plate detector DIP6040 (Bruker AXS). All data sets were collected at a cryogenic temperature of 100 K. SPR analysis The interaction between RamR and each substrate was analysed by SPR spectroscopy with a Biacore T200 biosensor instrument (GE Healthcare). RamR was immobilized onto flow cells in a CM5 sensor chip using an amine-coupling method. Binding analyses were carried out at 25 °C and a flow rate of 30 μl min −1 . Substrates in running buffer (1 × PBS, 3 mM DTT and 5% dimethylsulphoxide, pH 7.4) were run over the RamR at several concentrations as indicated. An empty flow cell, without any immobilized protein, was used as a reference. The binding curves were analysed using the steady-state affinity analysis supplied with the BIA evaluation software (GE Healthcare). To analyse the interaction of RamR with the ramA operator, the 5′-biotinylated 100-bp DNA fragment of the ramR–ramA intergenic region, as well as the 100-bp control fragment of the gyrB gene, was immobilized onto a SA sensor chip (GE Healthcare). Binding analyses were carried out at 25 °C and at a flow rate of 30 μl min −1 . The RamR protein was diluted in the running buffer (10 mM HEPES, 150 mM NaCl, 1 mM EDTA and 0.05% vol/vol Surfactant P20, pH 7.4) and injected over the sensor surface in two replicates for 2 min. To analyse the inhibitory effect of substrates on the DNA-binding affinity of RamR, drugs at several concentrations, as indicated, were injected with 250 nM RamR for 2 min. The data were normalized by subtracting the response from a control DNA-immobilized flow cell. Dissociation was recorded for 2 min. Regeneration of the surfaces was performed with 10 mM Tris and 2 M NaCl for 30 s followed by washes for 2 min. The inhibition caused by substrates was calculated by comparing the binding of particular RamR to DNA with and without substrates. Electrophoretic mobility shift assay The DNA probe used for EMSA, which contained the ramR–ramA intergenic region, was amplified by PCR using the Platinum PCR SuperMix High Fidelity (Invitrogen) and primers ramRA _PR_100F and ramRA _PR_100R ( Supplementary Table S5 ). The amplified 100-bp DNA fragment was purified using the Qiaquick PCR Purification Kit (Qiagen) and was labelled with digoxigenin (DIG) using a DIG gel shift kit 2nd generation (Roche Diagnostics). A total volume of 11 μl EMSA reaction mixture contained 15.5 fmol labelled DNA and 0, 15, 20, 25 or 30 pmol purified RamR in the binding buffer (20 mM Tris-HCl (pH 8.0), 200 mM NaCl and 3 mM DTT). To test the inhibitory effect of drugs on the DNA-binding affinity of RamR, each drug was added in the EMSA reaction mixture as indicated. After 15 min at room temperature, the samples were loaded onto 6% nondenaturing acrylamide gels, electrophoresed in electrophoresis buffer (0.5 × Tris-buffered EDTA buffer and 2% glycerol) and transferred onto a positively charged nylon membrane (Roche). The bands revealed by the DIG gel shift kit were visualized with an LAS-3000 (Fujifilm). Gene expression analysis using β-galactosidase assays Single colonies of NES84 strain to be assayed were inoculated into 2 ml of LB containing the appropriate antibiotics. After overnight incubation at 37 °C, cultures were diluted 1:50 in LB medium and then incubated at 37 °C for 5 h. To examine the effect of the drugs on ramA expression, each drug was added to secondary cultures at the following concentrations: 2 mM ethidium bromide, 0.1 mM dequalinium, 1 mM rhodamine 6G, 0.2 mM crystal violet and 2 mM berberine. β-Galactosidase activities were determined as described by Miller [25] All assays were performed in triplicate. Accession codes: The coordinates for unliganded RamR, and the RamR–berberine, RamR–crystal violet, RamR–dequalinium, RamR–ethidium bromide and RamR–rhodamine 6G complexes, have been deposited in the Protein Data Bank under accession numbers 3VVX , 3VW2 , 3VW1 , 3VW0 , 3VVY and 3VVZ , respectively. How to cite this article: Yamasaki, S. et al. The crystal structure of multidrug-resistance regulator RamR with multiple drugs. Nat. Commun. 4:2078 doi: 10.1038/ncomms3078 (2013).